Advancing plant phenology and reduced herbivore production in a terrestrial system associated with sea ice decline The contribution of declining Arctic sea ice to warming in the region through Arctic amplification suggests that sea ice decline has the potential to influence ecological dynamics in terrestrial Arctic systems. Empirical evidence for such effects is limited, however, particularly at the local population and community levels. Here we identify an Arctic sea ice signal in the annual timing of vegetation emergence at an inland tundra system in West Greenland. According to the time series analyses presented here, an ongoing advance in plant phenology at this site is attributable to the accelerating decline in Arctic sea ice, and contributes to declining large herbivore reproductive performance via trophic mismatch. Arctic-wide sea ice metrics consistently outperform other regional and local abiotic variables in models characterizing these dynamics, implicating large-scale Arctic sea ice decline as a potentially important, albeit indirect, contributor to local-scale ecological dynamics on land. Rising atmospheric CO 2 concentrations and sea ice loss have contributed to a rate of warming in the Arctic nearly double that at lower latitudes [1] , [2] , [3] , [4] , [5] . The accelerating seasonal decline in sea ice extent [6] , [7] ( Fig. 1 ), concentration [4] and thickness [8] , [9] in the Arctic [10] interacts with atmospheric and oceanic forcings via ice-albedo and ice-insulation feedbacks to amplify regional warming and stimulate further ice loss [4] . The main focus of ecological repercussions of projected sea ice loss has been on pagophillic species, whose dynamics have already been perturbed by diminishing sea ice cover [3] , [5] , [11] , [12] , [13] , [14] , [15] , [16] . In contrast, indirect weather-mediated effects of continued ice loss on terrestrial species are less clear. 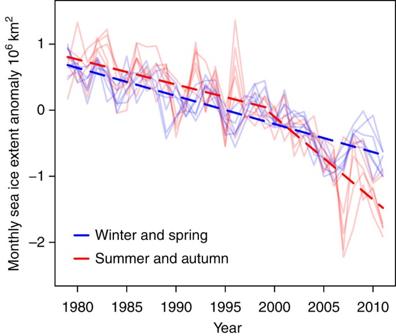Figure 1: Monthly Arctic sea ice extent index anomalies. Anomalies calculated from 1979 to 2011 mean are colour coded by season (winter and spring: December–May; summer and autumn: June–November). The rate of decline in monthly Arctic sea ice extent over this time period increased significantly in the summer and autumn months (red dashed) beginning in 2000 (95% confidence interval: 1997–2002). Figure 1: Monthly Arctic sea ice extent index anomalies. Anomalies calculated from 1979 to 2011 mean are colour coded by season (winter and spring: December–May; summer and autumn: June–November). The rate of decline in monthly Arctic sea ice extent over this time period increased significantly in the summer and autumn months (red dashed) beginning in 2000 (95% confidence interval: 1997–2002). Full size image Evidence for near coastal warming associated with regional sea ice decline is widely reported [17] , [18] , [19] , [20] , but broad-scale sea ice and temperature feedbacks also contribute to terrestrial warming not associated with coastal advection [17] , [21] . Empirical support for a role of sea ice in terrestrial ecological dynamics has thus far been limited to remotely sensed indices of vegetation productivity measured at moderate (500 m) to coarse (12 km) spatial grains along coastal regions [18] , [19] . These studies, in combination with modelling and heuristic arguments [21] , [22] , draw primary focus to the indirect ecosystem-level responses of terrestrial systems to sea ice loss. Less well-documented so far are local-scale effects and those affecting the dynamics of ecological populations and communities, especially those far from the coast, despite long-standing acknowledgement of their importance [23] , [24] . Here we investigate the potential for an Arctic sea ice signal in the local-scale dynamics at two trophic levels of an inland, mountainous tundra study system (67.11°N 50.34°W) near Kangerlussuaq in Low-Arctic West Greenland [25] , [26] , [27] using data derived from an ongoing, long-term observational study of ecological responses to climate change [28] , [29] . We explore the explanatory power of regional and Arctic-wide sea ice dynamics alongside other broad- and local-scale measures of climate variability in relation to the interannual variation in the timing of plant growth and the timing of parturition and reproductive performance of a migratory caribou ( Rangifer tarandus ) population. Our results suggest that sea ice decline is an important driver of the timing of the plant-growing season and trophic mismatch with caribou at this study site. Recent Arctic sea ice decline Annual sea ice extent over the Arctic has exhibited negative trends across all months from 1979 to 2011 ( Fig. 1 ). Time series of monthly Arctic sea ice extent aggregated by summer, and fall months exhibited a significant change towards more rapid sea ice decline around the year 2000 (95% confidence interval: 1997, 2002; the Davies test, k =30, P <0.001), but no significant aggregate acceleration in sea ice loss was detectable in winter and spring (the Davies test, k =30, P =0.17). Drivers of plant phenology The annual date of the midpoint of the plant-growing season at the study site, that of 50% species emergence, advanced from 2002 to 2011 ( Fig. 2 ; triangles, solid black line) by 1.6±0.53 days per year or ~16 days (linear regression R 2 =0.53, n =10, F(1,8)=8.977, P =0.02). Local temperature was a poor predictor of the date of 50% emergence in all years (best-fit regression models—local monthly temperature (May): R 2 =0.23, n =10, F(1,8)=2.421, P =0.16; Fig. 3a ; Local Summer Warmth Index year t : R 2 =0.33, n =10, F(1,8)=3.997, P =0.08; Fig. 3b ; local thawing degree days (TDD): R 2 =0.27, n =9 (2011 subdaily temperatures unavailable), F(1,7)=2.618, P =0.15). In contrast, monthly Arctic-wide sea ice extent (ASIE) from winter (January or February) and early summer (June) was a strong predictor of both interannual variation and the trend in dates of 50% plant species emergence ( R 2 =0.80 ( Figs 2a,b and 3c ) and 0.83 ( Fig. 2a,b ), respectively; n =10, F(2,7)=14.01, 17.62, P <0.004). Large-scale temperature and regional sea ice cover closest to the study area (Davis Strait/Baffin Bay) were also poor predictors of the annual date of 50% emergence at the site (best-fit regression models—Davis Strait/Baffin Bay Ice Cover (June): R 2 =0.08, n =9, F(1,7)=0.621, P =0.45; Fig. 3d ; Arctic Summer Warmth Index year t−1 : R 2 =0.26, n =10, F(1,8)=2.785, P =0.13; Fig. 3e ; Arctic-wide monthly surface temperature (April): R 2 =0.28, n =10, F(1,8)=3.055, P =0.12; Fig. 3f ), despite the expected stronger correlation between regional, rather than Arctic-wide, sea ice and local temperature in the months leading up to plant emergence ( Fig. 4a,b ). 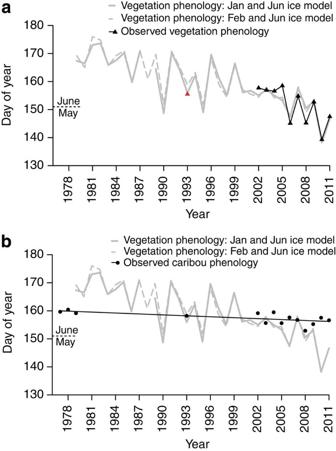Figure 2: Long-term differential response between trophic levels to diminishing Arctic sea ice. (a) Time series of observed (black triangles, black line) and predicted (grey lines) timing of 50% plant species emergence at the study site near Kangerlussuaq, Greenland, based on January (or February) and June multiple regression (y=β0+β1Jan(or Feb)E+β2JunE+ε, wherey=day of year of 50% plant species emergence in yeart, Jan(or Feb)E=January (or February) Arctic-wide sea ice extent (106km2) in yeart, JunE=June Arctic-wide sea ice extent (km2) in yeart). 1993 (red triangle) was not included in the parameterization of the model, but is plotted inato show the minimal difference between observed and predicted values for that year. The gap in the January- and June-modelled phenology series reflects a gap in the satellite-based sea ice extent record (1988). (b) Observed dates of 50% caribou calves born at the study site near Kangerlussuaq, Greenland (black circles, solid black regression line) plotted over the same phenology models asa. These time series document a divergence in the phenologies of caribou and the plant community in recent years, but also demonstrate a sustained flip in the timing of plant growth relative to herbivore parturition since the year 2000, a change driven primarily by earlier plant phenology relative to the comparatively fixed timing of caribou calving. Figure 2: Long-term differential response between trophic levels to diminishing Arctic sea ice. ( a ) Time series of observed (black triangles, black line) and predicted (grey lines) timing of 50% plant species emergence at the study site near Kangerlussuaq, Greenland, based on January (or February) and June multiple regression ( y = β 0 + β 1 Jan(or Feb)E+ β 2 JunE+ ε , where y =day of year of 50% plant species emergence in year t , Jan(or Feb)E=January (or February) Arctic-wide sea ice extent (10 6 km 2 ) in year t , JunE=June Arctic-wide sea ice extent (km 2 ) in year t ). 1993 (red triangle) was not included in the parameterization of the model, but is plotted in a to show the minimal difference between observed and predicted values for that year. The gap in the January- and June-modelled phenology series reflects a gap in the satellite-based sea ice extent record (1988). ( b ) Observed dates of 50% caribou calves born at the study site near Kangerlussuaq, Greenland (black circles, solid black regression line) plotted over the same phenology models as a . These time series document a divergence in the phenologies of caribou and the plant community in recent years, but also demonstrate a sustained flip in the timing of plant growth relative to herbivore parturition since the year 2000, a change driven primarily by earlier plant phenology relative to the comparatively fixed timing of caribou calving. 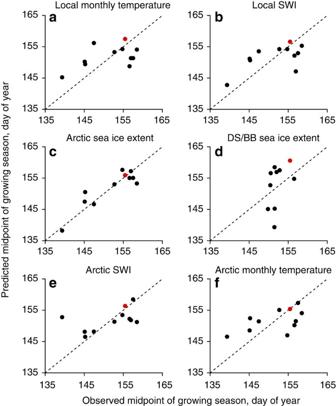Figure 3: Vegetation phenology models informed by temperature and sea ice metrics at local and broad scales. Each panel depicts the best-fit phenology model for a temporal or spatial scale of abiotic predictor(s). Predicted values of the timing of 50% plant species emergence are plotted against observed values from the study site. Model fits are organized in rows by local temperature (top row—two temporal scales), sea ice cover (centre row—two spatial scales) and Arctic-wide temperature (bottom row—two temporal scales). The dashed line in each panel depicts the 1:1 relationship between predicted and observed values. All panels used models parameterized with data from 2002 to 2011 (black circles) exceptdwhere no 2011 data were yet available. Red circles represent data from 1993 not used in the model parameterization. Abiotic predictors identified for each best-fit model scale are as follows: (a) May mean monthly temperature from Kangerlussuaq, Greenland; (b) Kangerlussuaq, Greenland Summer Warmth Index (SWI) (that is, thawing degree months) in the (The parentheses usage in this legend is inconsistent when referring to each panel. Panel d should have parenthesis when it is referred to for the second time in this legend (as it is being defined here) but not in the first reference in this panel) current year of plant emergence; (c) January and June Arctic sea ice extent; (d) is the Davis Strait/Baffin Bay regional sea ice extent in June of the year of plant emergence; (e) Arctic-wide SWI of the year before plant emergence; (f) April Arctic-wide mean monthly temperature. Full size image Figure 3: Vegetation phenology models informed by temperature and sea ice metrics at local and broad scales. Each panel depicts the best-fit phenology model for a temporal or spatial scale of abiotic predictor(s). Predicted values of the timing of 50% plant species emergence are plotted against observed values from the study site. Model fits are organized in rows by local temperature (top row—two temporal scales), sea ice cover (centre row—two spatial scales) and Arctic-wide temperature (bottom row—two temporal scales). The dashed line in each panel depicts the 1:1 relationship between predicted and observed values. All panels used models parameterized with data from 2002 to 2011 (black circles) except d where no 2011 data were yet available. Red circles represent data from 1993 not used in the model parameterization. Abiotic predictors identified for each best-fit model scale are as follows: ( a ) May mean monthly temperature from Kangerlussuaq, Greenland; ( b ) Kangerlussuaq, Greenland Summer Warmth Index (SWI) (that is, thawing degree months) in the (The parentheses usage in this legend is inconsistent when referring to each panel. Panel d should have parenthesis when it is referred to for the second time in this legend (as it is being defined here) but not in the first reference in this panel) current year of plant emergence; ( c ) January and June Arctic sea ice extent; ( d ) is the Davis Strait/Baffin Bay regional sea ice extent in June of the year of plant emergence; ( e ) Arctic-wide SWI of the year before plant emergence; ( f ) April Arctic-wide mean monthly temperature. 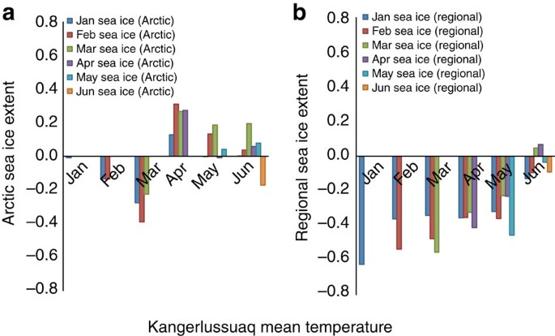Figure 4: Correlations between sea ice and inland temperature. Pearson’srcorrelation coefficients between linearly detrended local mean monthly temperature near the study site in Kangerlussuaq, Greenland and (a) ASIE or (b) regional Baffin Bay/Davis Strait sea ice extent. Correlations between ice extents from the months that precede each monthly mean temperature value are included for the calendar year up to and including June, the month when caribou calving and midpoint of the plant-growing season occurs. Full size image Figure 4: Correlations between sea ice and inland temperature. Pearson’s r correlation coefficients between linearly detrended local mean monthly temperature near the study site in Kangerlussuaq, Greenland and ( a ) ASIE or ( b ) regional Baffin Bay/Davis Strait sea ice extent. Correlations between ice extents from the months that precede each monthly mean temperature value are included for the calendar year up to and including June, the month when caribou calving and midpoint of the plant-growing season occurs. Full size image The explanatory power of the relationship between ASIE and local-scale plant phenology at the site remained high when all time series were detrended by year ( R 2 =0.66 (January and June ASIE) and 0.73 (February and June ASIE), respectively; n =10, F(2,7)=6.65 and 9.60, P <0.025). The mean error (±1 s.e.) between observed and predicted dates of 50% emergence was 2.08 (±0.55) days over the length of the observed time series, a smaller temporal range than the sampling resolution of most remote sensing and observer-based data series of plant phenology [30] . Hindcasting trophic mismatch A hindcast of the timing of plant emergence at the site using the Arctic-wide monthly sea ice model (January or February and June ASIE) suggests a trend over the past three decades towards earlier plant phenology at the study site (February and June model: β Plants =−0.741±0.099, R 2 =0.64, n =33; F(1,31)=55.78, P <0.001, dashed grey line; Fig 2a,b ). The observed date of 50% emergence in 1993, the earliest year plant phenology was recorded at this site [25] , was accurately predicted by our models ( Fig. 3a ; red triangle, 1993). Notably, this date was not used to parameterize either model. In contrast to the modelled time series of plant phenology, the observed timing of calving by caribou at the study site displayed little interannual variability ( Fig. 2b ; black circles) and only a slight rate of advance over the 33-year span of the data series ( β Caribou =−0.114±0.036, R 2 =0.45, n =14, F(1,12)=9.978, P =0.008; Fig. 2b ), obtained using observations from an earlier study [31] . This pattern is consistent with earlier reports based on 6 and 7 years of observational data on the timing of parturition by caribou in this population at the same site [16] , [29] . Increasing early mortality of caribou calves and declining production of calves in this population are related to increasing trophic mismatch driven by advancing plant phenology at this site ( Fig. 5a,b ). The relationship between plant phenology and the magnitude of trophic mismatch indicates that the earlier green-up occurs the stronger is the mismatch in that year (Pearson’s r =−0.81, n =11, P =0.002; Fig. 5c ). A trophic mismatch index constructed using sea ice-modelled plant emergence data and empirical caribou calving data closely tracks our empirical index of trophic mismatch (Pearson’s r =0.70, n =11, P =0.02; Fig. 5d ) and indicates a strong trophic match in 1979 ( Fig. 5a,b ), a result that is consistent with earlier reports of caribou calf production at the study site in that year [31] . 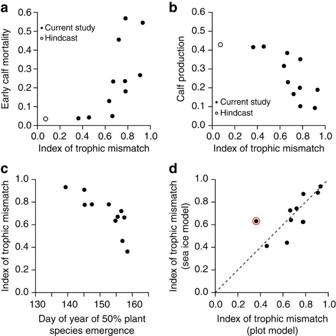Figure 5: Reproductive consequences of trophic mismatch. (a,b) The relationships between the magnitude of trophic mismatch, that is, the percentage of plant species emergent at the date of 50% caribou calves born, and early calf mortality (a) or caribou calf production (b) at the study site. Filled circles were calculated using data from the 11 years of the authors’ long-term observational study, whereas open circles depict empirical records of caribou reproductive performance from 1979 in relation to sea ice-informed estimates of trophic mismatch in that year. The lack of satellite-derived sea ice data before 1979 prevented the inclusion of the caribou data from 1977 and 1978 that are shown inFig. 2b. (c) The relationship between the observed trophic mismatch index and observed dates of 50% plant species emergence at the study site. Earlier plant emergence results in increasing mismatch with the timing of offspring production by caribou, a period of critically high resource demand28,29,44. (d) Relationship between the original trophic mismatch index derived from plot-based vegetation phenology and the trophic mismatch index derived from a sea ice-only model estimate of vegetation phenology. The year 2005, circled in red, was characterized by a severe caterpillar outbreak27, when plant phenology was anomalously delayed by defoliation, resulting in lower plot-derived mismatch in that year. Figure 5: Reproductive consequences of trophic mismatch. ( a , b ) The relationships between the magnitude of trophic mismatch, that is, the percentage of plant species emergent at the date of 50% caribou calves born, and early calf mortality ( a ) or caribou calf production ( b ) at the study site. Filled circles were calculated using data from the 11 years of the authors’ long-term observational study, whereas open circles depict empirical records of caribou reproductive performance from 1979 in relation to sea ice-informed estimates of trophic mismatch in that year. The lack of satellite-derived sea ice data before 1979 prevented the inclusion of the caribou data from 1977 and 1978 that are shown in Fig. 2b . ( c ) The relationship between the observed trophic mismatch index and observed dates of 50% plant species emergence at the study site. Earlier plant emergence results in increasing mismatch with the timing of offspring production by caribou, a period of critically high resource demand [28] , [29] , [44] . ( d ) Relationship between the original trophic mismatch index derived from plot-based vegetation phenology and the trophic mismatch index derived from a sea ice-only model estimate of vegetation phenology. The year 2005, circled in red, was characterized by a severe caterpillar outbreak [27] , when plant phenology was anomalously delayed by defoliation, resulting in lower plot-derived mismatch in that year. Full size image Several lines of evidence suggest that the complex interaction between plant phenology and herbivore demographics is ostensibly driven by Arctic sea ice decline. First, there is a strong association between ASIE and plant phenology at our site ( Fig. 2 ). Second, before the acceleration of summer and autumn sea ice loss that began around the year 2000, the timing of 50% plant species emergence coincided with or followed, on average, the timing of caribou parturition at the site ( Fig. 2b ), contributing to greater trophic match (lower mismatch), lower offspring mortality and higher offspring production ( Fig. 5a,b ). Since the acceleration of summer and autumn sea ice loss began, however, plant phenology has shifted towards increasingly earlier 50% emergence, which now, on average, precedes caribou parturition ( Fig. 2b ). This, in turn, has exacerbated the previously documented trophic mismatch [28] , [29] , further reducing herbivore reproductive performance ( Fig. 5a,b ). Third, and finally, our estimates of annual trophic mismatch derived from observational plant phenology data ( Fig. 5a–c ) are accurately reproduced by an index of trophic mismatch that is constructed with sea ice extent-modelled plant phenology data ( Fig. 5d ). Although other large-scale and regional forcings, like Arctic surface temperature and nearby sea ice cover, are correlated with ASIE during some periods of the year [32] , they are poor or inconsistent predictors of annual dates of 50% plant species emergence at this site ( Fig. 3a,b,d–f ). The fact that ASIE outperformed even local predictors (TDD and Fig. 3a,b,d ) raises questions about the specific indirect mechanism(s) by which sea ice affects plant phenology that we cannot resolve with certainty, given the current data set. The phenomenon of large-scale integrative variables outperforming local-scale predictors in explanatory power is, however, well-documented in ecological studies [33] , [34] , and is particularly relevant to the relationship between plant phenology and sea ice. Arctic-wide sea ice influences many elements of climate variation at regional and local scales [35] , [36] , [37] , [38] , [39] , and plant phenology is driven by a complex interaction between many of these abiotic factors and the biotic environment integrated over a period of several months [40] . Isolating the mechanistic influence of a specific time window or single abiotic factor on these dynamics will require, at a minimum, spatially and/or temporally replicated local-scale phenology and productivity data that, at present, are rare. As the product of correlative analyses, our results share a limitation common to other efforts to assign attribution in ecological responses to climate change [41] , [42] . Recognizing this limitation is important, but not by default disqualifying [43] . Our results strongly suggest that interannual variability and the long-term decline in Arctic sea ice cover can have important indirect consequences for highly localized ecological dynamics, and complex interactions deriving from them, in terrestrial systems. Whereas such consequences are comparatively well-known, and more obviously expected, in marine systems [13] , our results highlight the need for greater focus on the indirect implications of sea ice loss for the dynamics and conservation of terrestrial species. Plant phenology Plant phenology data used in these analyses were derived from near-daily observations from early May to late June from 2002 to 2011 of all species emergent on 12 (0.5 m 2 ) permanently marked plots at three sites with differing aspects and elevations (260–300 m) [28] , [29] , [44] . Data from 1993 were collected using identical methods on a separate set of plots covering the same extent and elevational gradient within the study site [25] . The annual date of 50% of plant species emergence (hereafter in methods, 50% emergence) was calculated from nonlinear regression models fit to the across-plot-averaged time series of the percentage of species observed on each plot on day x in year y relative to the total number of species observed on each plot by the end of June in year y (refs 25 , 28 , 45 ). Herbivore phenology and demographics Caribou abundance, demographics and reproductive phenology were monitored at the study site and at the adjacent calving area over the same time period and at the same frequency as the vegetation phenology plots [25] , [28] . Caribou calving phenology was calculated using Caughley’s Indirect Method A [46] modified for use in wild populations [47] . Reproductive performance of the caribou population was calculated from changes in calving season demographics derived from near-daily observations of calf to population ratios excluding males. We defined calf production as the proportion of calves to the sum of calves and cows in the population in late June. Annual calf mortality was defined as the end of June proportion of calves to the sum of calves and cows divided by the peak proportion of calves to the sum of calves and cows observed during that season. These methods are consistent with those described in greater detail in previous reports from this site [25] , [28] , [44] . Sea ice The monthly ASIE index and monthly regional sea ice extent data for the Davis Strait/Baffin Bay area were obtained from the National Snow and Ice Data Center for January 1979 through December 2011/2010, respectively [48] , [49] . These gridded (25 km × 25 km) data series quantify the extent cover (all grid cells >0.15% sea ice cover multiplied by grid cell area) of sea ice as measured from a suite of satellite-based passive microwave sensors for the entire Arctic and the Davis Strait/Baffin Bay region (region graphically defined in ref. 50 ). Monthly ASIE anomalies were calculated based on 1979–2011 monthly means. These data were separated into two groups: the months leading up to and including the onset of terrestrial primary productivity (winter through spring: December to May) and the months of peak primary productivity and senescence (summer through autumn: June through November) to examine the implications of non-uniform ice loss throughout the year using the phenology of primary productivity as a yardstick. To identify the presence and timing of a significant acceleration in the rate of ice loss in these grouped sea ice time series, we applied a Davies test ( k =30) using the ‘segmented’ package in R (refs 51 , 52 ). This tests for the ‘best’ value at which a significant difference in slope can be identified through the use of naive Wald statistics corrected for repeated testing across ‘ k ’ evenly spaced potential break points [51] . Temperature Hourly (1999–2010) and mean monthly temperature (1978–2011) records for the village of Kangerlussuaq, Greenland (<25 km from study site) were obtained from the Danish Meteorological Institute [53] . TDD were calculated from the hourly data consistent with method 2 from McMaster and Wilhelm [54] . Accumulated TDD for each day of the year (DOY) were then calculated for 2002–2010. Local mean monthly temperature data were used to calculate the Summer Warmth Index (SWI) for the study site. The SWI is the sum of the mean monthly temperatures above zero (°C per month), effectively a measure of thawing degree months. Mean monthly Arctic-wide (65° N–90° N) surface temperatures were acquired from NCEP Reanalysis-derived data [55] provided by the NOAA/OAR/ESRL PSD, Boulder Colorado, USA ( http://www.esrl.noaa.gov/psd/ ). Relating inland temperatures to sea ice extent To explore the possibility of immediate and lagged influence of Arctic-wide and regional sea ice extent on Kangerlussuaq temperature, correlational analyses (Pearson’s r ) were run on linearly detrended monthly time series of local temperature and ASIE and Davis Strait/Baffin Bay sea ice extent. Results were used to guide model selection and interpretation for models linking sea ice with temperature and sea ice with plant phenology. Relating temperature to plant phenology We used linear regression to explore the effect of accumulated TDD year t on the DOY 50% emergence year t as well as effect of accumulated TDD by June 1 year t on DOY of 50% emergence year t . Linear regression was also used to relate local monthly mean temperatures to DOY of 50% emergence, the SWI of current and the previous summer to the DOY of 50% emergence and mean monthly temperatures and Arctic-wide SWI to DOY of 50% emergence. Relating inland plant phenology to sea ice extent Sea ice extent (ASIE and regional) was related to DOY of 50% emergence using linear regression models parameterized with 2002–2011 phenology data. The best candidate models were then confronted with 1993 phenology data to assess the error between predicted and observed values for a date outside the continuous sampling period. To isolate the influence of trend from interannual variability, the best-fit regressions were reanalyzed with detrended (by year) phenology and sea ice data. Relating caribou offspring production to plant phenology The synchrony of caribou calving phenology was related to plant phenology using the index of trophic mismatch developed previously [28] . This index is calculated, using a fitted logistic curve, as the percentage of plant species emergent on the date of 50% caribou births, and thus represents a measure of the state of forage plant resource availability midway through the season of herbivore parturition, a life history period with a critical influence on reproductive performance [28] . The annual values of this index were then regressed against end of season caribou calf production and early caribou calf mortality for 1993, 2002–2011, respectively, updating previous analyses [28] , [29] . Data on caribou calving from 1977 to 1979 were obtained from an earlier study that was conducted at the same study site by a different group using equivalent methods [31] . Relating caribou offspring production to sea ice extent Nonlinear logistic models were fit to sea ice-based estimates of plant phenology (15, 25, 40, 50, 60, 75 and 85% plant species emergent) for 1979, 1993 and 2002–2011 using the same methods detailed above for estimating the date of 50% species emergent. We then used these model coefficients (minimum coefficient of determination for all models was 0.68) to calculate the percent of the total number of plant species emergent on the date of observed 50% caribou births, effectively allowing for the calculation of a trophic mismatch index [28] solely using sea ice extent and caribou phenology data. This allowed for similar caribou productivity and mortality regressions against trophic mismatch as detailed above. All statistical analyses were conducted using the base package in the R statistical computing environment unless otherwise noted [52] . Throughout, best-fit regression models were identified using an information theoretics approach, specifically Akaike’s Information Criterion corrected for small sample sizes (AICc). Models were considered equivalent if ΔAIC<2. How to cite this article: Kerby, J. T. et al . Advancing plant phenology and reduced herbivore production in a terrestrial system associated with sea ice decline. Nat. Commun. 4:2514 doi: 10.1038/ncomms3514 (2013).